Spiracular air breathing in polypterid fishes and its implications for aerial respiration in stem tetrapods The polypterids (bichirs and ropefish) are extant basal actinopterygian (ray-finned) fishes that breathe air and share similarities with extant lobe-finned sarcopterygians (lungfishes and tetrapods) in lung structure. They are also similar to some fossil sarcopterygians, including stem tetrapods, in having large paired openings (spiracles) on top of their head. The role of spiracles in polypterid respiration has been unclear, with early reports suggesting that polypterids could inhale air through the spiracles, while later reports have largely dismissed such observations. Here we resolve the 100-year-old mystery by presenting structural, behavioural, video, kinematic and pressure data that show spiracle-mediated aspiration accounts for up to 93% of all air breaths in four species of Polypterus . Similarity in the size and position of polypterid spiracles with those of some stem tetrapods suggests that spiracular air breathing may have been an important respiratory strategy during the fish-tetrapod transition from water to land. Fish spiracles are paired tubes extending from the dorsal surface of the skull into the buccopharyngeal chamber. They are a plesiomorphic character of gnathostomes formed during embryonic development of the jaws when the vestige of the first gill cleft is reduced in size by the anterior migration of the second (hyoid-hyomandibular) arch to support the jaws (mandibular arch) [1] , [2] . Among extant fishes, spiracles are common in elasmobranchs (sharks and rays) where, in addition to sensory functions, they sustain mouth-bypassing ventilatory flow to the gills when the subterminal mouth is obstructed by substrate or engaged in prey manipulation [2] , [3] , [4] . A few extant early-diverging actinopterygian lineages (Polypteriformes (bichirs and ropefish) and Acipenseriformes (sturgeons and paddlefish)) have spiracles, but only the polypterids, a freshwater African family (~11 species of Polypterus and the monotypic Erpetoichthys ) have spiracles large enough to significantly aid in respiration [4] , [5] , [6] , [7] . Polypterids respire bimodally (both aquatically and aerially); they breathe air using ventrally paired lungs with a glottal valve and a pulmonary circulation remarkably similar to that of lungfish and tetrapods [8] , [9] , [10] , [11] , [12] . Polypterid lungs are typically ventilated by recoil aspiration [13] , [14] . Exhalation begins with the contraction of muscles within the lung wall that ejects air into the buccopharyngeal chamber from where it is forced out the opercula. Polypterids have a stiff body wall formed by thick, overlapping ganoid scales, and with lung compression, a negative internal pressure (−530 to −800 Pa) is established within the body cavity and the body wall collapses inward. The aspiration of air occurs when the glottal valve opens, the stiff body wall recoils and subambient pressure draws air into the lungs [13] . Air entry into polypterid lungs has long been regarded to occur through the mouth [7] , [13] , [14] , [15] . However, observations from over a century ago indicated the occurrence of spiracular inhalation with the ‘mouth submerged’ and ‘spiracles widely opened above the surface of the water (with) a sound produced as of the sucking of air [16] .’ A similar report later stated that Polypterus could ‘rapidly inhale air through its spiracles by emerging the dorsal part of its body [17] .’ However, these observations were not systematically studied, proved hard to verify and had subsequently been discounted, ‘(polypterids) do not, as others have suggested, breathe through the spiracles [13] .’ Here we clarify these discrepancies by providing the first definitive evidence of spiracle-mediated aspiration occurring in Polypterus . The description of spiracular air breathing in this extant fish group provides a mechanistic model for examining the role and potential use of the large and similarly positioned spiracles of stem tetrapods. Spiracular air breathing and spiracle morphology Confirmation of spiracular air breathing in Polypterus was based on structural, behavioural, kinematic and pressure data, including observations made on four species ( P. delhezi , P. lapradei , P. ornatipinnis and P. senegalus ) taking 732 breaths over 343 h. Hinged dermal bones or ossicles on the skull roof ( Fig. 1a–c ) serve as valves that seal the spiracles, except when opened briefly during aspiration ( Fig. 1d ). High-resolution magnetic resonance images show these valves and the spiracle’s route along the lateral wall of the braincase to the buccopharyngeal chamber ( Fig. 1a,b ). 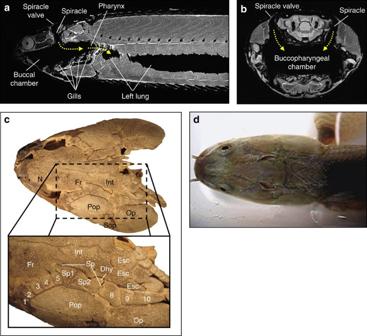Figure 1: Morphology associated withPolypterusspiracular air breathing. (a,b) Sagittal and transverse magnetic resonance images ofP. palmasshowing the path (arrows) of air through the spiracles to the buccopharyngeal chamber and lungs. (c) Dorsal view of the head ofP. bichirshowing the position of the two dermal ossicles (Sp1, Sp2) that form the spiracular valve (Sp). (d)P. delheziwith the spiracular valves open and emerged during aspiration. Dhy, dermohyal; Esc, extrascapular bone; Fr, frontal; Int, Intertemporosupratemporal bone; N, nasal; Op, opercle; Pop, preopercle; Sop, subopercle. Non-spiracular ossicles are labelled with numbers: prespiracular ossicles (1–5), post-spiracular ossicles (8–10). Figure 1: Morphology associated with Polypterus spiracular air breathing. ( a , b ) Sagittal and transverse magnetic resonance images of P. palmas showing the path (arrows) of air through the spiracles to the buccopharyngeal chamber and lungs. ( c ) Dorsal view of the head of P. bichir showing the position of the two dermal ossicles (Sp1, Sp2) that form the spiracular valve (Sp). ( d ) P. delhezi with the spiracular valves open and emerged during aspiration. Dhy, dermohyal; Esc, extrascapular bone; Fr, frontal; Int, Intertemporosupratemporal bone; N, nasal; Op, opercle; Pop, preopercle; Sop, subopercle. Non-spiracular ossicles are labelled with numbers: prespiracular ossicles (1–5), post-spiracular ossicles (8–10). Full size image Kinematics of spiracular air breathing Video analysis ( Fig. 2 and Supplementary Movies 1–3 ) reveal the sequential kinematic stages of spiracular air breathing ( Fig. 3 ), which begins when the fish aligns with the water surface and emerges the upper region of its head bordering the spiracles ( Fig. 2a ). There is a decrease in dorsal–ventral body diameter as ejected lung gas moves into the buccopharyngeal chamber, which subsequently expands ( Fig. 2b ). While the buccopharyngeal chamber expands, exhaled air begins to leave the opercular slits ( Fig. 2b ) and is completely cleared as the buccopharyngeal chamber subsequently compresses ( Fig. 2c ). Exhalation is rapidly followed by the opening and extension of the dermal spiracle valves above the water surface ( Fig. 2d ) and the aspiration of fresh air into the lungs. During aspiration, the buccopharyngeal chamber also expands ( Fig. 2d ), and following the closure of the spiracular valves, the lungs are ‘topped off’ by the compression of the buccal force pump ( Fig. 2e ). Finally, air remaining in the buccopharyngeal chamber is cleared out of the opercular openings following resumption of aquatic ventilation ( Fig. 2f ). 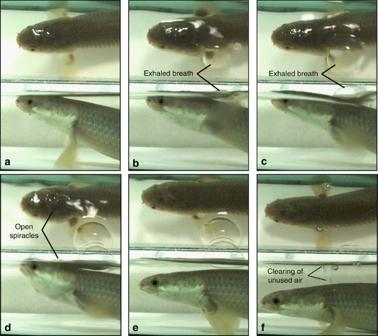Figure 2: Video images showing the key stages in the spiracular air-breath cycle forP. senegalus. (a) Head reaches and becomes parallel to the water surface. (b) Dorsal–ventral body diameter posterior of the pectoral fins is reduced with the ejection of air from the lungs into the buccopharyngeal chamber (which expands) and out the opercula. (c) Compression of the buccopharyngeal and opercular chambers expels additional lung air out the opercular openings. (d) The spiracular valves open above the water surface resulting in air aspiration into the buccopharyngeal chamber (which expands) and lungs (as indicated by an increase in dorsal–ventral body diameter). (e) Spiracular valve closure is rapidly followed by the compression of the buccopharyngeal chamber, which forces additional air into the lungs, further expanding dorsal–ventral body diameter. (f) As the fish leaves the surface, the gills are ventilated with water, which clears unused air from the buccopharyngeal chamber out the opercular slits. (SeeSupplementary Movie 3for complete footage associated with these still images). Figure 2: Video images showing the key stages in the spiracular air-breath cycle for P. senegalus . ( a ) Head reaches and becomes parallel to the water surface. ( b ) Dorsal–ventral body diameter posterior of the pectoral fins is reduced with the ejection of air from the lungs into the buccopharyngeal chamber (which expands) and out the opercula. ( c ) Compression of the buccopharyngeal and opercular chambers expels additional lung air out the opercular openings. ( d ) The spiracular valves open above the water surface resulting in air aspiration into the buccopharyngeal chamber (which expands) and lungs (as indicated by an increase in dorsal–ventral body diameter). ( e ) Spiracular valve closure is rapidly followed by the compression of the buccopharyngeal chamber, which forces additional air into the lungs, further expanding dorsal–ventral body diameter. ( f ) As the fish leaves the surface, the gills are ventilated with water, which clears unused air from the buccopharyngeal chamber out the opercular slits. (See Supplementary Movie 3 for complete footage associated with these still images). 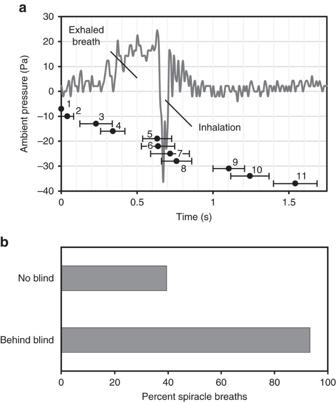Figure 3: Spiracle use inPolypterusair breathing. (a) Kinematic events during spiracular air breathing inP. delhezi(numbered black dots, means±s.d.) in relation to the pressure oscillation in a 70-ml closed air chamber showing an initial pressure rise caused by air-breath release followed by an abrupt pressure drop during the onset of inhalation. Kinematic events: (1) Body wall begins to compress as air is forced out of the lungs (time=0); (2) Buccopharyngeal chamber begins to expand; (3) Exhaled breath begins to leave the opercular openings; (4) Buccopharyngeal chamber begins to compress to force additional air out the opecula; (5) Spiracles open; (6) Exhaled breath has completely left the opercula; (7) Body diameter begins to increase as air is drawn in through the spiracles and enters the lungs through recoil aspiration; (8) Buccopharyngeal chamber begins to expand drawing air entering the spiracles into the buccopharyngeal chamber; (9) Spiracles close; (10) Buccopharyngeal chamber begins to compress forcing additional air into the lungs; (11) Buccopharyngeal chamber compression ends signaling the end of lung inflation. Kinematic events are the mean of 20 analysed air breaths; for visual simplicity only a single representative pressure trace is shown. (b) Percentage of total air breaths taken through the spiracles for fourPolypterusspecies without a blind (190 air breaths observed) and behind a blind (542 air breaths observed). Full size image Figure 3: Spiracle use in Polypterus air breathing. ( a ) Kinematic events during spiracular air breathing in P. delhezi (numbered black dots, means±s.d.) in relation to the pressure oscillation in a 70-ml closed air chamber showing an initial pressure rise caused by air-breath release followed by an abrupt pressure drop during the onset of inhalation. Kinematic events: (1) Body wall begins to compress as air is forced out of the lungs (time=0); (2) Buccopharyngeal chamber begins to expand; (3) Exhaled breath begins to leave the opercular openings; (4) Buccopharyngeal chamber begins to compress to force additional air out the opecula; (5) Spiracles open; (6) Exhaled breath has completely left the opercula; (7) Body diameter begins to increase as air is drawn in through the spiracles and enters the lungs through recoil aspiration; (8) Buccopharyngeal chamber begins to expand drawing air entering the spiracles into the buccopharyngeal chamber; (9) Spiracles close; (10) Buccopharyngeal chamber begins to compress forcing additional air into the lungs; (11) Buccopharyngeal chamber compression ends signaling the end of lung inflation. Kinematic events are the mean of 20 analysed air breaths; for visual simplicity only a single representative pressure trace is shown. ( b ) Percentage of total air breaths taken through the spiracles for four Polypterus species without a blind (190 air breaths observed) and behind a blind (542 air breaths observed). Full size image Pressure measurements and mouth versus spiracular inhalation The synchronizing of kinematic data with ambient pressure measurements made on Polypterus during spiracular air breathing in a small chamber ( Fig. 3a , pressure positive during expiration, negative during the onset of aspiration) confirms the use of recoil aspiration similar to that previously described using the mouth [13] . In addition, our results solve the long-standing mystery [7] , [8] , [13] , [14] , [15] , [16] , [17] of mouth versus spiracular aspiration by showing that the spiracles were used for 93% of air breaths when the fish was filmed from behind a blind (which decreased fish wariness and stress), but when the blind was removed (and the fish could see the observer), the spiracles were only used 40% of the time ( Fig. 3b ). It is thus our interpretation that the preferred Polypterus air-breathing mode is through the spiracles and that stress or other factors common in a laboratory setting may encourage mouth inhalation, which in our observations, often involved a rapid dash to and from the surface ( Supplementary Movie 4 ) as opposed to the more stealthy, but prolonged, process of aligning the spiracles with the air–water interface ( Supplementary Movies 1–3 ). Our confirmation of spiracle-aided recoil aspiration in polypterids documents the first-known occurrence of the transformation of spiracles from water conduits to the gills to air conduits to the lungs. This appears to be an adaptation for life in shallow freshwater habitats where hypoxia is common and requires the use of aerial respiration [8] , [9] , [18] . Polypterids are commonly found in hypoxic swamps, lakes and stagnant pools and tributaries of northern and central Africa’s major river basins [18] . In these habitats, aspiration through short airways on the dorsal surface of the skull is efficacious in water too shallow to incline the body sufficiently to raise the mouth above the surface to take a breath. When placed in very shallow water, our observations suggest that Polypterus has difficulty raising the mouth above the water surface and is therefore reliant upon the spiracles to breathe air. Spiracular inhalation is likely advantageous in allowing the head to remain in the water, thereby limiting changes in body orientation and contributing to shallow water swimming efficiency, increased stealth during foraging and enabling the eyes to remain submerged (resulting in an uninterrupted view of the surrounding aquatic environment during the air breath). Confirmation of spiracular air breathing in Polypterus allows for speculation into the role of the mysteriously large spiracles of stem tetrapods from the Devonian (~380 million years ago). Like Polypterus ( Fig. 4a ), stem tetrapods, which were also almost certainly bimodal (lung and gill) breathers [19] , [20] , [21] , [22] , were thought to inhabit shallow freshwater habitats including shallow pools, water edges, oxbow lakes, channels and other marginal aquatic environments in which stagnation and hypoxia would have been prevalent [20] , [21] , [22] and spiracular air breathing advantageous. The stem tetrapods shown in Fig. 4b–d ( Gogonasus [23] , Tiktaalik [24] , Ventastega [25] ) resemble Polypterus in having pronounced spiracles located high on the head that are consistent with spiracular air breathing. Stem tetrapod skull morphology ( Fig. 4b–d ) differs from that of their predecessors for which this region is well preserved ( Fig. 4e–g ) by having an elongate snout and a short posterior region, with a relatively reduced otic capsule and a rearward shifted and larger spiracular opening, becoming a ‘V’-shaped spiracular notch (also termed the otic or temporal notch or cleft) [20] . The spiracular chamber of the stem tetrapods shown in Fig. 4 (and others such as Panderichthys ) is further defined by a ridge on the inner surface of the entopterygopid, indicating that the spiracles slanted posteroventrally to the throat region where the opening for lungs would have been located [23] , [26] . 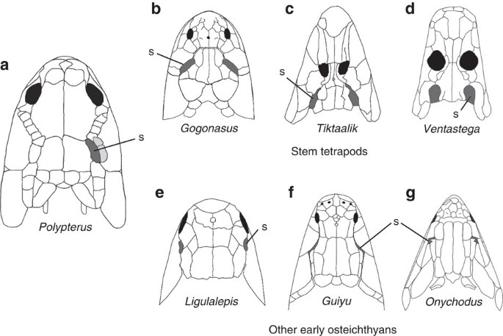Figure 4: Dorsal view of the skull ofPolypterusin comparison to three stem tetrapods and three other early osteichthyans. (a)Polypterus. (b)Gogonasus23. (c)Tiktaalik24. (d)Ventastega25. (e)Ligulalepis(modified from Basdenet al.27). (f)Guiyu(reconstructed based on study material from Zhuet al.28). (g)Onychodus29.Polypterusis shown with both the spiracular valve closed (left) and open (right). Figure 4: Dorsal view of the skull of Polypterus in comparison to three stem tetrapods and three other early osteichthyans. ( a ) Polypterus . ( b ) Gogonasus [23] . ( c ) Tiktaalik [24] . ( d ) Ventastega [25] . ( e ) Ligulalepis (modified from Basden et al. [27] ). ( f ) Guiyu (reconstructed based on study material from Zhu et al. [28] ). ( g ) Onychodus [29] . Polypterus is shown with both the spiracular valve closed (left) and open (right). Full size image While previous studies have speculated on the association of the large spiracles in tetrapods with aquatic [26] or aerial ventilation [20] , our observations on Polypterus provide, for the first time, a mechanistic model for the plausible use of spiracle-mediated air breathing in members of this lineage. Many stem tetrapods had thick, highly articulated and overlapping peg-and-socket-like rhombic scales [21] , [22] , [23] , [24] , [25] that could have allowed for lung ventilation via recoil aspiration in a manner similar to Polypterus . However, the use of the buccal pump in Polypterus to deliver spiracle-derived air to the lungs at the end of the air-breath cycle suggests that other mechanisms to move air through the spiracles may be possible and thus large, interlaced scales and the use of recoil respiration are not necessarily prerequisites for this air-breathing mode. Unlike Polypterus , in which spiracular air breathing allows the laterally positioned eyes to remain underwater, the eyes of later stem tetrapods such as Tiktaalik [24] and Ventastega [25] ( Fig. 4c,d ) were located high on the dorsal surface of the skull. Spiracular air breathing in these animals would have thus likely forced the eyes above the water surface and may have allowed them to take a crocodilian-like approach to stalking terrestrial prey at the water–land interface. Our results support the idea that spiracle-aided aspiration may have been an integral step in the vertebrate transition to land with early stem tetrapods using their large and dorsally located spiracles for air intake near the shoreline. Subsequent changes to their pectoral and pelvic girdles, limb development, and a suite of other anatomical adaptations, including the transformation of the spiracular region for sound transmittance and reception, prepared later tetrapods for a successful invasion of the terrestrial environment [19] , [21] , [24] , [25] , [26] . Animal care and husbandry All Polypterus observation, care, husbandry and experimentation were conducted in accordance with Protocol S00080 of the University of California, San Diego Institutional Animal Care and Use Committee. Video analyses of breathing mode and cycle A Sony HDR-UX7 high-definition, high-speed capacity video camera was used to document fish breathing patterns and the air-breath cycle for four Polypterus specimens from four species ( P . delhezi , 29.7 cm; P . lapradei , 21.2 cm; P . ornatipinnis 29.4 cm; P. senegalus , 19.8 cm). Three hundred forty-three hours of observations were obtained for fish placed in an 80-l aquarium fitted with a partition that confined the fish to the front third (60.0 × 11.0 × 30.0 cm, length × width × height) for filming while still allowing sufficient space to swim freely. At the start of most observation periods, additional heaters in the tank were turned on and N 2 gas was bubbled into the system to reduce the dissolved O 2 level and increase air-breath frequency (all breath observation data were obtained at water temperatures between 24 and 33 °C with dissolved O 2 levels ranging from air saturation to zero). For each observation period, the number of breaths the fish took and the percentage of these that involved inhalation via the spiracles or mouth were recorded. In spiracular breaths, the mouth remained closed below the water surface and the spiracle valves opened into the air. Mouth air breaths usually involved a rapid rush to the surface that emerged the head and mouth. In order to assess fish ‘wariness’ on air-breathing mode (spiracle versus mouth), Polypterus were observed with the aquarium placed behind a blind so that the fish could not see the observer or out into the room and with the aquarium open so that the fish could see the observer. Some observations were also made on fish in a very shallow aquarium (37 × 8 × 6.5 cm) with a mirror set at 45° to allow simultaneous side and dorsal views (for example, Fig. 2 ). Video-based breath cycle analyses were made for each of the four species and included the temporal logging of the key events consistently occurring during each breath. Ambient pressure associated with spiracular breathing To measure external air pressure fluctuations associated with Polypterus spiracular air-breathing, fish were placed in an air-tight triangular prism aquarium (45 × 25 × 26 cm) with a small pocket of air (70 ml) at the top apical end. A 2F Millar pressure transducer (MICRO-CATH 825-0101, Millar Instruments, Houston, TX, USA) connected to an amplifier (PCU-2000, Millar Instruments) and interfaced to a digital-analog acquisition system (DI-220, DATAQ Instruments, Akron, OH, USA) was placed in the air phase and synchronized with high-speed video to document an initial pressure rise (during exhalation) and subsequent drop (associated with inhalation) during the Polypterus air-breath cycle. Magnetic resonance imaging Data were acquired from a formalin-fixed P . palmas (26.0 cm) that was exposed to 2.5 mM l −1 solution of gadolinium-based MR contrast agent ProHance (gadoteridol: Bracco Diagnostics, Princeton, NJ, USA) in phosphate-buffered saline and 0.01% sodium azide for ~3 weeks prior to imaging. Equilibration in this contrast agent achieves a significant reduction in longitudinal relaxation time ( T 1 ) and a corresponding increase in MR signal-to-noise. The specimen was scanned with a 7 T (300 MHz) small animal scanner (Bruker Biospec Avance II, Bruker AXS Inc., Madison, WI, USA), consisting of a 210-mm horizontal bore magnet equipped with a shielded gradient set to an inner diameter of 90 mm, and a maximum gradient strength of 630 m T m −1 , maximum slew rate 6,300 T m −1 s −1 and rise time 160 μs, using a 35-mm diameter circular polarized 1H-radio frequency linear transmit/receive birdcage volume coil (Bruker Biospin GmbH, Ettlingen, Germany). Data were collected using T 1 /T 2 -weighted 3D fast low-angle shot (FLASH) GRE acquisition pulse sequence in the transverse plane at 100 μm 3 isotropic voxel resolution with the following parameters: 15° flip angle, 25.9 ms repetition time, 12.9 ms echo time, 300 kHz bandwidth, 35 × 70 × 30 mm in-field field-of-view and 10 averages. Data were converted to DICOM ( http://medical.nema.org/ ) format for image processing and visualization. How to cite this article: Graham, J. B. et al. Spiracular air breathing in polypterid fishes and its implications for aerial respiration in stem tetrapods. Nat. Commun. 5:3022 doi: 10.1038/ncomms4022 (2014).